An IL-27/NFIL3 signalling axis drives Tim-3 and IL-10 expression and T-cell dysfunction The inhibitory receptor T-cell immunoglobulin and mucin domain-3 (Tim-3) has emerged as a critical regulator of the T-cell dysfunction that develops in chronic viral infections and cancers. However, little is known regarding the signalling pathways that drive Tim-3 expression. Here, we demonstrate that interleukin (IL)-27 induces nuclear factor, interleukin 3 regulated (NFIL3), which promotes permissive chromatin remodelling of the Tim-3 locus and induces Tim-3 expression together with the immunosuppressive cytokine IL-10. We further show that the IL-27/NFIL3 signalling axis is crucial for the induction of Tim-3 in vivo . IL-27-conditioned T helper 1 cells exhibit reduced effector function and are poor mediators of intestinal inflammation. This inhibitory effect is NFIL3 dependent. In contrast, tumour-infiltrating lymphocytes from IL-27R −/− mice exhibit reduced NFIL3, less Tim-3 expression and failure to develop dysfunctional phenotype, resulting in better tumour growth control. Thus, our data identify an IL-27/NFIL3 signalling axis as a key regulator of effector T-cell responses via induction of Tim-3, IL-10 and T-cell dysfunction. T-cell immunoglobulin and mucin domain-3 (Tim-3) was initially identified as an inhibitory receptor expressed on interferon (IFN)-γ-producing CD4 + (T helper 1 (Th1)) and CD8 + T (Tc1) cells [1] . Interaction between Tim-3 and its ligand, galectin-9, was shown to suppress effector T-cell function resulting in Tim-3-dependent cell death during autoimmune tissue inflammation [2] . Exciting new research has demonstrated that Tim-3 is a key regulator of the exhausted antigen-specific CD4 + and CD8 + T cells that arise in both humans and mice during chronic viral infections, such as HIV, hepatitis C virus (HCV), hepatitis B virus and lymphocytic choriomeningitis virus (LCMV) [3] , [4] , [5] and in cancer [6] , [7] , [8] . Exhaustion refers to a state of dysfunction that typically arises in a hierarchical manner whereby effector T cells first lose the ability to proliferate and be cytotoxic in response to antigen stimulation. This is then followed by the loss of interleukin (IL)-2 secretion, which is followed by a gradual loss of tumour-necrosis factor (TNF) and IFN-γ and increased production of the immunosuppressive cytokine IL-10. Accordingly, exhausted T cells pose a significant barrier to the induction of productive anti-viral or anti-tumour immunity. In contrast, one could envisage that in autoimmune diseases, the induction of T-cell exhaustion would be beneficial. Although primarily studied in CD8 + T cells, exhaustion also occurs in CD4 + T cells [3] . Exhausted T cells are characterized by their sustained expression of inhibitory receptors. Programmed death-1 (PD-1) was the first such molecule to be identified; its inhibitory function is essential for the induction of T-cell exhaustion during chronic LCMV infection in mice, and during chronic HIV infection in humans [9] , [10] , [11] , [12] . It is now appreciated that co-expression of PD-1 with other inhibitory receptors, such as Tim-3, contributes to the induction of T-cell exhaustion and as such defines T cells with more deeply exhausted phenotype [5] . Importantly, simultaneous blockade of the Tim-3 and PD-1 signalling pathways restores cytotoxic T lymphocyte function and cytokine production, whereas blockade of the PD-1 pathway alone is less effective. Thus, targeting Tim-3 on exhausted T cells provides a potential therapeutic avenue for treating multiple chronic viral infections and cancers. On the other hand, increasing Tim-3 expression would be beneficial for autoimmunity as reduced amounts of Tim-3 expression have been associated with a number of human autoimmune diseases [13] . In spite of the increasing data linking Tim-3 to the suppression of T-cell immunity, little is known about the signals by which its expression is induced on T cells. It was therefore important to identify the cytokines and pathways that induce the expression of this inhibitory molecule. In this study, we demonstrate that IL-27, an immunosuppressive cytokine, is a potent inducer of Tim-3 expression on T cells. IL-27 strongly induces the expression of the transcription factor nuclear factor, interleukin 3 regulated (NFIL3), which cooperates with T-bet, to induce the expression of Tim-3 and IL-10. In addition, IL-27-conditioned Th1 cells exhibited poor effector function and are poor mediators of intestinal inflammation in an NFIL3-dependent manner. We show that IL-27 signalling is required for the induction of Tim-3 + exhausted T cells and promotion of tumour growth. Thus, we have uncovered that an IL-27/NFIL3 signalling axis drives inhibition of effector T cells via the induction of Tim-3, IL-10 and dysfunctional T-cell phenotype. IL-27 is a potent inducer of Tim-3 in naïve CD4 + T cells Our previous study indicated that T-bet is more functionally critical than signal transducer and activator of transcription 4 (STAT4) in the induction of Tim-3 expression on Th1 cells [14] . The modest reduction of Tim-3 expression in IL-12-polarized STAT4 −/− Th1 cells indicated that Tim-3 expression is not completely dependent on IL-12 signalling. To further explore other cytokines with potential to induce Tim-3, we tested a panel of cytokines for their ability to induce Tim-3 expression on naïve CD4 + T cells. After analysing Tim-3 transcription by real-time PCR, we observed that IL-27 was the most potent inducer of Tim-3 transcription ( Fig. 1a ). Indeed, IL-27 was more potent than IL-12, which only slightly increased Tim-3 transcription over that observed in the control neutral (Th0) condition ( Fig. 1a ). 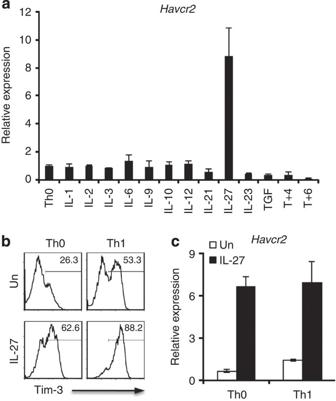Figure 1: IL-27 induces Tim-3 expression. (a) Naïve CD4 T cells were activated by anti-CD3 and anti-CD8 antibodies in the presence of different cytokines. After 72 h of activation, cells were harvested for quantitative PCR (qPCR) analysis of Tim-3 (Havcr2) transcription. Havcr2 expression was normalized to that of β-actin. (b,c) Naïve CD4+T cells were activated with anti-CD3 and anti-CD28 antibodies under neutral (Th0) or Th1 (IL-12 treatment) conditions with or without IL-27. To analyse Tim-3 protein expression, the cells were restimulated with anti-CD3 and anti-CD28 antibodies on day 5 for 24 h before examination of Tim-3 expression by flow cytometry (c). The transcription ofTim-3 (Havcr2)was examined by qPCR 72 h after activation (b). Data are representative of at least three independent experiments with similar results (a,b: mean±s.d.). Un, Untreated; IL-27, IL-27-treated. Figure 1: IL-27 induces Tim-3 expression. ( a ) Naïve CD4 T cells were activated by anti-CD3 and anti-CD8 antibodies in the presence of different cytokines. After 72 h of activation, cells were harvested for quantitative PCR (qPCR) analysis of Tim-3 (Havcr2) transcription. Havcr2 expression was normalized to that of β-actin. ( b , c ) Naïve CD4 + T cells were activated with anti-CD3 and anti-CD28 antibodies under neutral (Th0) or Th1 (IL-12 treatment) conditions with or without IL-27. To analyse Tim-3 protein expression, the cells were restimulated with anti-CD3 and anti-CD28 antibodies on day 5 for 24 h before examination of Tim-3 expression by flow cytometry ( c ). The transcription of Tim-3 (Havcr2) was examined by qPCR 72 h after activation ( b ). Data are representative of at least three independent experiments with similar results ( a , b : mean±s.d.). Un, Untreated; IL-27, IL-27-treated. Full size image As Tim-3 expression is upregulated during Th1 differentiation [1] , we asked whether IL-27 further enhances Tim-3 expression on differentiating Th1 cells. We therefore activated naïve CD4 + T cells under Th0 or Th1 (with IL-12) conditions in the presence or absence of IL-27, and observed that IL-27-treated T cells (Th0+IL-27) exhibited higher Tim-3 protein expression than cells cultured with IL-12 alone (Th1 condition). Importantly, addition of IL-27 to differentiating Th1 cells (Th1+IL-27) exhibited an additive effect and induced the most Tim-3 protein expression ( Fig. 1b ). Similarly, we found that IL-27 had a dominant effect on Tim-3 mRNA induction in both conditions ( Fig. 1c ). IL-27-induced NFIL3 and T-bet regulates both Tim-3 and IL-10 IL-27 has been shown to induce IL-10-producing Tr1 cells, which are a key component of IL-27-mediated immunosuppression [15] , [16] . Accordingly, we examined whether IL-27 would induce IL-10 together with Tim-3 in activated T cells. We therefore examined IL-10 expression in Th0 and Th1 cells treated with IL-27 and found that IL-27 potentiated the induction of IL-10 under both conditions ( Fig. 2a ). We further found that IL-27 induced IL-10 together with Tim-3 as a significant fraction of IL-27-treated cells co-expressed with Tim-3 and IL-10 ( Fig. 2b ). Similarly, IL-27 could induce Tim-3 and IL-10 expression in CD8 + T cells in both neutral (Tc0) and Tc1 (with IL-12) conditions ( Supplementary Fig. 1 ). Examination of the kinetics of Tim-3 and IL-10 expression during IL-27 stimulation revealed that both Tim-3 and IL-10 transcription are induced with similar kinetics ( Fig. 2c ), suggesting a common transcriptional programme for their induction. 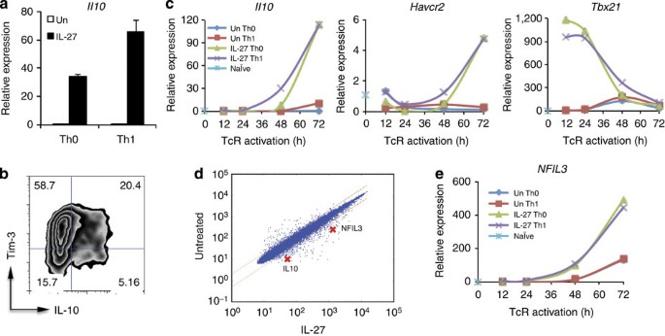Figure 2: An IL-27-induced NFIL3 and T-bet regulate the expression of both Tim-3 and IL-10. Naïve CD4+T cells were differentiated under Th0 or Th1 (by IL-12 treatment) condition with or without IL-27. (a) IL-10 (Il10) mRNA expression was detected by qPCR 72 h after TcR activation (mean± s.d.). (b) To detect Tim-3 and IL-10 co-expression in IL-27-treated Th1 cells, the cells were restimulated with anti-CD3 and anti-CD28 antibodies on day 5 after TcR activation for 24 h before subjected to flow cytometry analysis. (c,e) Naïve CD4+T cells were activated with anti-CD3 and anti-CD28 antibodies under Th0 or Th1 culture condition with or without IL-27. RNA was isolated at 12, 24, 48 and 72 h after TcR activation for qPCR to determine the expression kinetics of IL-10, Tim-3, T-bet (Tbx21) and NFIL3. Data are representative of at least three independent experiments with similar results. (d) Gene profile studies. Naïve CD4+T cells from C57BL/6 mice were stimulated with anti-CD3 and anti-CD28 antibodies in the presence of IL-27 for 60 h. The cells were subjected to gene profile analysis. The scatter plot represents comparative transcriptome analysis between cells under neutral culture condition and cells treated with IL-27. Figure 2: An IL-27-induced NFIL3 and T-bet regulate the expression of both Tim-3 and IL-10. Naïve CD4 + T cells were differentiated under Th0 or Th1 (by IL-12 treatment) condition with or without IL-27. ( a ) IL-10 ( Il10 ) mRNA expression was detected by qPCR 72 h after TcR activation (mean± s.d.). ( b ) To detect Tim-3 and IL-10 co-expression in IL-27-treated Th1 cells, the cells were restimulated with anti-CD3 and anti-CD28 antibodies on day 5 after TcR activation for 24 h before subjected to flow cytometry analysis. ( c , e ) Naïve CD4 + T cells were activated with anti-CD3 and anti-CD28 antibodies under Th0 or Th1 culture condition with or without IL-27. RNA was isolated at 12, 24, 48 and 72 h after TcR activation for qPCR to determine the expression kinetics of IL-10, Tim-3, T-bet (Tbx21) and NFIL3. Data are representative of at least three independent experiments with similar results. ( d ) Gene profile studies. Naïve CD4 + T cells from C57BL/6 mice were stimulated with anti-CD3 and anti-CD28 antibodies in the presence of IL-27 for 60 h. The cells were subjected to gene profile analysis. The scatter plot represents comparative transcriptome analysis between cells under neutral culture condition and cells treated with IL-27. Full size image It is known that IL-27 induces T-bet [17] , a transcription factor that has a role in both Tim-3 and IL-10 expression [14] , [18] , [19] . However, overexpression of T-bet alone in T cells under different experimental settings does not always increase Tim-3 expression [14] , [19] , indicating that maximal levels of Tim-3 and IL-10 expression in IL-27-treated Th1 cells may not be due to the induction of T-bet alone and that other transcription factors must be required for optimal Tim-3 transcription. Indeed, close examination of the kinetics of IL-27-induced T-bet transcription revealed that T-bet mRNA levels peaked within 24 h of T-cell activation and gradually declined thereafter. In contrast, Tim-3 and IL-10 transcription gradually increased until peaking at 72 h at which time T-bet transcription had declined to near basal levels similar to that observed in Th0 cells ( Fig. 2c ). This decline of T-bet transcription before Tim-3 and IL-10 transcription indicates that other transcription factor(s) must be required for sustained induction of Tim-3 and IL-10 transcription. We therefore undertook gene expression profiling of naïve CD4 + T cells stimulated in the presence or absence of IL-27 at eight different time points in order to elucidate the IL-27-induced transcription network in CD4 + T cells. With this information, we built a transcriptional network that could identify transcription factors based on their kinetics and by labelling each edge with a time stamp to identify a connection between a regulator and its target [20] . Through this analysis, we identified that NFIL3 was a transcription factor whose transcription was highly induced by IL-27 ( Fig. 2d, e and Supplementary Fig. 2 ). Indeed, NFIL3 has been found to be essential for IL-10 expression in Th1 cells [21] . Importantly, the expression kinetics of NFIL3 mRNA paralleled that of IL-10 and Tim-3 expression ( Fig. 2c,e ), thus raising the possibility that NFIL3 may be the transcription factor that mediates IL-27-driven expression of Tim-3 and IL-10. NFIL3 is induced in both exhausted and anergic T cells Given the association of both Tim-3 and IL-10 expression with T-cell exhaustion and the indication that NFIL3 may drive Tim-3 and IL-10 expression, we examined the expression of NFIL3 in exhausted T cells. Indeed, we found that NFIL3 is induced to much higher levels in virus-specific CD8 + T cells in mice infected with the chronic clone-13 (Clone 13) strain of LCMV compared with virus-specific CD8 + T cells in mice infected by the Armstrong (Arm) strain. In addition, we found that NFIL3 is upregulated in ionomycin-induced anergic T cells ( Supplementary Fig. 3a,b ), which also upregulate Tim-3 ( Supplementary Fig. 3c ). Taken together, these data support that NFIL3, a transcription factor that is highly induced by IL-27 signalling, may represent a key regulator of Tim-3 expression and the induction of T-cell dysfunction. NFIL3 is critical for the expression of Tim-3 and IL-10 To confirm the role of NFIL3 in the regulation of Tim-3 and IL-10, we cultured naïve wild-type ( WT ) and NFIL3 −/− CD4 + T cells in vitro under Th0 or Th1 conditions in the presence or absence of IL-27. We found that NFIL3 deficiency resulted in reduced Tim-3 and IL-10 expression in all conditions, suggesting that NFIL3 is critical for the expression of both Tim-3 and IL-10 ( Fig. 3a ). Importantly, when compared with IL-27-treated WT Th0 cells, IL-27-induced Tim-3 and IL-10 expression levels were largely abrogated in NFIL3 −/− Th0 cells. Tim-3 expression was similarly attenuated in NFIL3 −/− CD8 + T cells ( Supplementary Fig. 4 ). Together, these data suggested that NFIL3 is a critical transcription factor for IL-27-mediated Tim-3 expression. 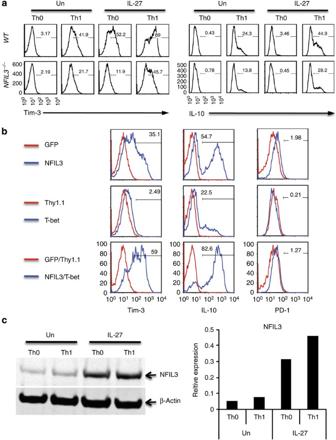Figure 3: IL-27-mediated Tim-3 expression is dependent on the functional cooperation between T-bet and NFIL3. (a) Naïve CD4+T cells from wild-type (WT) C56BL/6 mice andNFIL3−/−mice were activated with anti-CD3 and anti-CD28 under Th0 or Th1 (IL-12 treatment) condition with or without IL-27. Five days after TcR activation, cells were restimulated with anti-CD3 and anti-CD28 for 24 h and subjected to detection of the expression of Tim-3 and IL-10 by flow cytometry. (b) Naïve CD4+T cells were transduced with retrovirus carrying NFIL3 cDNA (NFIL3), T-bet cDNA (T-bet), or both NFIL3 and T-bet. Retrovirus empty vector-transduced T cells were used as controls (GFP for NFIL3, Thy1.1 for T-bet). Four days after TcR activation, the expression of Tim-3, IL-10 and PD-1 was examined by flow cytometry. The percentage represents the expression of Tim-3, IL-10 or PD-1 in NFIL3- or T-bet-transduced, or NFIL3/T-bet-co-transduced cells relative to GFP- or Thy1.1-expressing empty vector-transduced, or GFP/Thy1.1 empty vector-co-transduced cells, respectively. (c) Naïve CD4+T cells were activated by anti-CD3 and anti-CD28 under Th0 and Th1 condition (IL-12 treatment) with or without IL-27. Three days after TcR activation, the expression of NFIL3 expression was detected by western blot analysis (left) and its relative expression to β-actin was quantified by LI-COR Odyssey Imaging System (right). Data are representative of at least three independent experiments with similar results. Figure 3: IL-27-mediated Tim-3 expression is dependent on the functional cooperation between T-bet and NFIL3. ( a ) Naïve CD4 + T cells from wild-type ( WT ) C56BL/6 mice and NFIL3 −/− mice were activated with anti-CD3 and anti-CD28 under Th0 or Th1 (IL-12 treatment) condition with or without IL-27. Five days after TcR activation, cells were restimulated with anti-CD3 and anti-CD28 for 24 h and subjected to detection of the expression of Tim-3 and IL-10 by flow cytometry. ( b ) Naïve CD4 + T cells were transduced with retrovirus carrying NFIL3 cDNA (NFIL3), T-bet cDNA (T-bet), or both NFIL3 and T-bet. Retrovirus empty vector-transduced T cells were used as controls (GFP for NFIL3, Thy1.1 for T-bet). Four days after TcR activation, the expression of Tim-3, IL-10 and PD-1 was examined by flow cytometry. The percentage represents the expression of Tim-3, IL-10 or PD-1 in NFIL3- or T-bet-transduced, or NFIL3/T-bet-co-transduced cells relative to GFP- or Thy1.1-expressing empty vector-transduced, or GFP/Thy1.1 empty vector-co-transduced cells, respectively. ( c ) Naïve CD4 + T cells were activated by anti-CD3 and anti-CD28 under Th0 and Th1 condition (IL-12 treatment) with or without IL-27. Three days after TcR activation, the expression of NFIL3 expression was detected by western blot analysis (left) and its relative expression to β-actin was quantified by LI-COR Odyssey Imaging System (right). Data are representative of at least three independent experiments with similar results. Full size image To further examine the role of NFIL3 in the regulation of Tim-3 expression, we generated a retroviral expression construct for NFIL3 (NFIL3) and ectopically expressed NFIL3 in naïve CD4 + T cells. Compared with cells transduced with empty retroviral vector (green fluorescent protein (GFP)), overexpression of NFIL3 dramatically increased Tim-3 expression ( Fig. 3b ). This effect was highly specific for Tim-3 as NFIL3 only slightly increased the expression of other inhibitory receptors such as PD-1, LAG3 and CD160 ( Fig. 3b and Supplementary Fig. 5 ). We also analysed cytokine production and found that NFIL3-transduced cells exhibit significantly increased IL-10 expression ( Fig. 3b ). Although our data clearly show that NFIL3 induces Tim-3, the expression of Tim-3 expression is much higher on NFIL3-transduced cells cultured under Th1 conditions ( Supplementary Fig. 5 ), indicating a potential functional cooperation between NFIL3- and Th1-associated transcription factor(s). We therefore examined the transcriptional cooperation between NFIL3 and T-bet in the regulation of Tim-3 and IL-10 expression. We found that NFIL3 was much more potent in inducing both Tim-3 and IL-10 expression than T-bet. However, overexpression of both NFIL3 and T-bet synergistically enhanced both Tim-3 and IL-10 expression ( Fig. 3b ). The fact that overexpression of T-bet in Th0 cells only slightly enhances Tim-3 expression once again indicates that T-bet alone is not sufficient for optimal Tim-3 expression without significant induction of other transcription factors. Interestingly, neither NFIL3 nor T-bet significantly induced PD-1 expression ( Fig. 3b ). Thus, our data indicate a fundamental difference in the transcriptional regulation of PD-1 and Tim-3 expression. To determine whether IL-27-mediated induction of Tim-3 and IL-10 is also linked to its induction of NFIL3, we examined the amounts of NFIL3 protein in Th0 and Th1 cells in the presence or absence of IL-27 stimulation. A low level of NFIL3 protein was detected in Th0 cells, and no significant increase was found in Th1 cells. However, NFIL3 was strongly induced by IL-27 and this was further enhanced in IL-27-treated Th1 cells ( Fig. 3c and Supplementary Fig. 12a ). Thus, IL-27 promotes NFIL3 expression, which in turn activates Tim-3 and IL-10 expression. Mechanism of IL-27-induced Tim-3 and IL-10 expression STAT1 and STAT3 are two major transducers in the IL-27 signalling pathway. To determine whether IL-27-driven Tim-3 and IL-10 expression is dependent on either STAT1 or STAT3, we activated naive CD4 + T cells from STAT1 −/− and STAT3 fl/fl x CD4-Cre ( STAT3 cko ) mice in Th0 conditions or in the presence of either IL-12 or IL-27. We found that STAT1 −/− CD4 + T cells exhibited significant defects in both Tim-3 and IL-10 expression when compared with WT CD4 + T cells. This defect became more pronounced upon stimulation by either IL-27 or IL-12 ( Fig. 4a ). Interestingly, STAT3 deficiency did not affect Tim-3 or IL-10 expression in cells cultured under Th0 condition. However, IL-27-treated STAT3 cko CD4 + T cells clearly displayed reduced Tim-3 and IL-10 expression relative to WT cells. Surprisingly, this defect in Tim-3 and IL-10 expression was also observed in IL-12-treated cells, indicating a role for STAT3 in both IL-12- and IL-27-mediated Tim-3 and IL-10 expression ( Fig. 4b ). 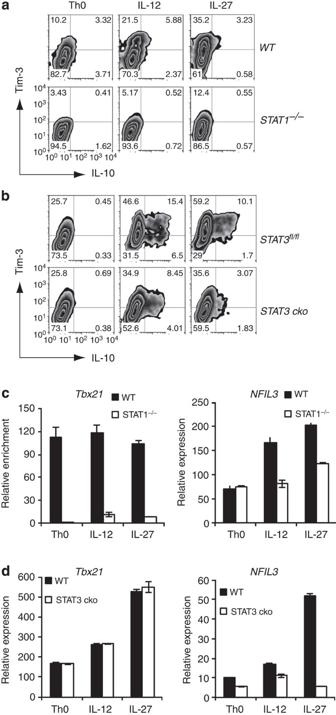Figure 4: STAT1/T-bet and STAT3/NFIL3 mediate IL-27-induced Tim-3, and IL-10, expression. (a,b) Naïve CD4+T cells purified fromSTAT1−/−mice (STAT1−/−) (a) orSTAT3fl/flx CD4-Cremice (STAT3 cko) (b) and their wild-type littermates (WTforSTAT1−/−andSTAT3fl/flforSTAT3 cko) were activated with anti-CD3 and anti-CD28 antibodies under neutral (Th0) condition, or under the stimulation of IL-12 or IL-27. Five days after activation, the cells were restimulated by anti-CD3 and anti-CD28 for 24 h and were subjected to the detection of Tim-3 and IL-10 by flow cytometry. (c,d) Naïve CD4+T cells as described inaandbwere stimulated with anti-CD3 and anti-CD28 antibodies for 72 h and were subjected to qPCR analysis for the transcription of T-bet (Tbx21) and NFIL3. The expression was normalized to the β-actin. Data are representative of at least two independent experiments with similar results (a,b: mean±s.d.). Figure 4: STAT1/T-bet and STAT3/NFIL3 mediate IL-27-induced Tim-3, and IL-10, expression. ( a , b ) Naïve CD4 + T cells purified from STAT1 −/− mice ( STAT1 −/− ) ( a ) or STAT3 fl/fl x CD4-Cre mice ( STAT3 cko ) ( b ) and their wild-type littermates ( WT for STAT1 −/− and STAT3 fl/fl for STAT3 cko ) were activated with anti-CD3 and anti-CD28 antibodies under neutral (Th0) condition, or under the stimulation of IL-12 or IL-27. Five days after activation, the cells were restimulated by anti-CD3 and anti-CD28 for 24 h and were subjected to the detection of Tim-3 and IL-10 by flow cytometry. ( c , d ) Naïve CD4 + T cells as described in a and b were stimulated with anti-CD3 and anti-CD28 antibodies for 72 h and were subjected to qPCR analysis for the transcription of T-bet (Tbx21) and NFIL3. The expression was normalized to the β-actin. Data are representative of at least two independent experiments with similar results ( a , b : mean±s.d.). Full size image We next examined T-bet and NFIL3 transcription in STAT1 −/− or STAT3 cko CD4 + T cells. The absence of STAT1, but not STAT3, resulted in a profound reduction of T-bet transcription in all conditions ( Fig. 4c,d ). This is consistent with previous data indicating that STAT1, but not STAT3, is essential for T-bet expression [22] . In contrast, STAT1 deficiency only resulted in a modest reduction in NFIL3 expression in IL-12- and IL-27-stimulated cells but not cells cultured in Th0 condition ( Fig. 4c ), indicating that STAT1 partially affects NFIL3 expression. Further, we found that STAT3-deficient T cells exhibited partially reduced NFIL3 transcription under Th0 condition and IL-12 treatment. Importantly, these STAT3-deficient T cells showed a near complete loss of IL-27-induced NFIL3 expression ( Fig. 4d ), indicating that STAT3 is essential for IL-27-induced NFIL3 transcription. Thus, IL-27 triggers two distinct and non-redundant pathways: a STAT1/T-bet and a STAT3/NFIL3 pathway, both of which are critical for the induction of Tim-3 and IL-10 expression in T cells. IL-27 directly induces Tim-3 expression via NFIL3 and T-bet To elucidate the molecular mechanism of IL-27-mediated activation of Tim-3 transcription, we performed chromatin immunoprecipitation (ChIP) assays to examine histone modification of the Tim-3 locus. The ChIP products were subjected to quantitative PCR (qPCR) using primer sets that cover the whole Tim-3 locus ( Fig. 5a and Supplementary Table 1 ). We examined histone H3 acetylation, a marker for permissive chromatin modification favouring gene expression, in chromatin samples prepared from Th0 cells and IL-27-treated Th1 cells. We found that IL-27-treated Th1 cells exhibited significantly higher enrichment of histone H3 acetylated at N-terminal lysine residues (H3Ac) in the proximal promoter region and in intron 1 of the Tim-3 locus ( Fig. 5b ). In addition, the same regions in the Tim-3 locus were also highly enriched with histone H3 trimethylation at lysine 4 (H3K4me3), another permissive chromatin modification marker ( Fig. 5c ). Together, these data indicate that IL-27 signalling promotes chromatin modifications in the Tim-3 locus that favour the transcription of Tim-3 mRNA in Th1 cells. 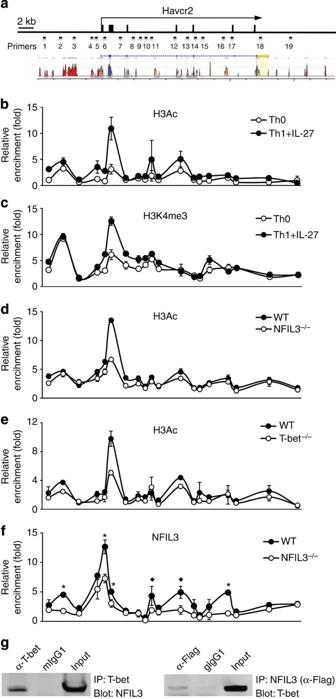Figure 5: IL-27-induced permissive chromatin modification in the Tim-3 locus is both NFIL3 and T-bet dependent. (a) Mouse Tim-3 locus and the location of PCR primers for ChIP-qPCR analysis. The histogram (derived from ECR Browser:http://www.dcode.org) represents CNSs which stand for 70% or greater identity over at least 100 bp stretches of the genomic DNA sequences between human and mouse Tim-3 locus (blue: coding exons, red: intergenic regions; orange: intronic regions; yellow: UTRs). ChIP-PCR primers were marked according to their relative location in the Tim-3 locus. (b,c) Naïve CD4+T cells from C57BL/6 mice were activated by anti-CD3 and anti-CD28 antibodies under Th0 or IL-27-treated Th1 condition. The cells were restimulated on day 5 for 24 h and were subjected to ChIP-qPCR for detection of H3Ac (b) and H3K4me3 (c) enrichment in the Tim-3 locus. (d,e) In a similar experimental setting, H3Ac enrichment in the Tim-3 locus was examined inNFIL3−/−CD4+T cells andT-bet−/−CD4+T cells. (f)NFIL3−/−andWTCD4+T cells were activated by anti-CD3 and anti-CD28 antibodies under Th1 culture condition in the presence of IL-27. Four days after T-cell activation, the cells were subjected to ChIP-qPCR to analyse NFIL3 enrichment in the Tim-3 locus. NFIL3-enriched areas marked with * represent the potential NFIL3-binding sites in both human and mouse homologous sequences, whereas those marked with ♦ represent the potential NFIL3-binding sites only in mouse sequences. (g) Expression plasmids for NFIL3 and T-bet were transiently transfected into 293T cells. Whole-cell lysates were harvested 48 h after transfection for co-IP to detect the interaction between NFIL3 and T-bet. Data are representative of at least two independent experiments with similar results (a–e: mean±s.d.). IP, immunoprecipitation. Figure 5: IL-27-induced permissive chromatin modification in the Tim-3 locus is both NFIL3 and T-bet dependent. ( a ) Mouse Tim-3 locus and the location of PCR primers for ChIP-qPCR analysis. The histogram (derived from ECR Browser: http://www.dcode.org ) represents CNSs which stand for 70% or greater identity over at least 100 bp stretches of the genomic DNA sequences between human and mouse Tim-3 locus (blue: coding exons, red: intergenic regions; orange: intronic regions; yellow: UTRs). ChIP-PCR primers were marked according to their relative location in the Tim-3 locus. ( b , c ) Naïve CD4 + T cells from C57BL/6 mice were activated by anti-CD3 and anti-CD28 antibodies under Th0 or IL-27-treated Th1 condition. The cells were restimulated on day 5 for 24 h and were subjected to ChIP-qPCR for detection of H3Ac ( b ) and H3K4me3 ( c ) enrichment in the Tim-3 locus. ( d , e ) In a similar experimental setting, H3Ac enrichment in the Tim-3 locus was examined in NFIL3 −/− CD4 + T cells and T-bet −/− CD4 + T cells. ( f ) NFIL3 −/− and WT CD4 + T cells were activated by anti-CD3 and anti-CD28 antibodies under Th1 culture condition in the presence of IL-27. Four days after T-cell activation, the cells were subjected to ChIP-qPCR to analyse NFIL3 enrichment in the Tim-3 locus. NFIL3-enriched areas marked with * represent the potential NFIL3-binding sites in both human and mouse homologous sequences, whereas those marked with ♦ represent the potential NFIL3-binding sites only in mouse sequences. ( g ) Expression plasmids for NFIL3 and T-bet were transiently transfected into 293T cells. Whole-cell lysates were harvested 48 h after transfection for co-IP to detect the interaction between NFIL3 and T-bet. Data are representative of at least two independent experiments with similar results ( a – e : mean±s.d.). IP, immunoprecipitation. Full size image To test whether NFIL3 is required for this permissive chromatin modification in the Tim-3 locus, we compared H3Ac enrichment in IL-27-treated Th1 cells derived from WT and NFIL3 −/− mice. The absence of NFIL3 resulted in profound attenuation of H3Ac enrichment in the proximal promoter region and intron1 ( Fig. 5d ). Interestingly, a similar reduction of H3Ac enrichment in the same region of the Tim-3 locus was also found in T-bet-deficient cells ( Fig. 5e ). Taken together, our data suggest T-bet and NFIL3 are both essential for IL-27-mediated permissive chromatin modification in the Tim-3 locus. Our previous ChIP-qPCR data demonstrated that T-bet binds to the Tim-3 proximal promoter region [14] , thus providing evidence supporting the direct involvement of T-bet in the chromatin remodelling of the Tim-3 locus. To identify whether NFIL3 directly binds to the Tim-3 locus, we conducted ChIP-qPCR using chromatin samples prepared from WT and IL-27-treated NFIL3 −/− Th1 cells and identified multiple NFIL3-binding regions scattered in the Tim-3 distal and proximal promoter regions and introns 3, 4 and 5 ( Fig. 5f ). We further assembled a high-resolution map of NFIL3 binding in the Tim-3 locus by performing NFIL3 ChIP-Seq and observed that NFIL3 binding in the Tim-3 locus is in line with our ChIP-qPCR data ( Supplementary Fig. 6a ). In addition, we analysed published T-bet ChIP-Seq in Th1 cells [23] (GSE33802). Interestingly, the alignment of T-bet and NFIL3 binding revealed a high degree of co-localization of these two transcription factors in the Tim-3 locus, particularly in the introns of Tim-3 , indicating that they occupy common cis -regulatory regions with very close proximity ( Supplementary Fig. 6a ). Importantly, we were able to confirm the ChIP-Seq-identified T-bet-binding sites to the Tim-3 locus by ChIP-qPCR further supporting the potential functional interaction between T-bet and NFIL3 ( Supplementary Fig. 6b ). Further, a similar co-localization of T-bet and NFIL3 is also found in the IL-10 locus ( Supplementary Fig. 6a ). Thus, the ChIP-Seq data provided preliminary evidence for T-bet–NFIL3 interaction and their functional cooperation in both Tim-3 and IL-10 expression. Interestingly, both T-bet and NFIL3 ChIP-Seq and ChIP-qPCR results indicate stronger binding in the intragenic regions than in the proximal promoter region of the Tim-3 locus ( Fig. 5f and Supplementary Fig. 6a,b ), suggesting that T-bet and NFIL3 may function to optimize Tim-3 transcription through permissive chromatin modification of the Tim-3 locus. Indeed, we did not observe strong transcriptional activity from either transcription factors in driving Tim-3 promoter-luciferase reporter activity ( Supplementary Fig. 6d ). Given that NFIL3- and T-bet-binding sites are co-localized in multiple regions in the Tim-3 locus, we hypothesized that NFIL3 and T-bet may physically interact with each other to coordinate Tim-3 transcription. To test this hypothesis, we performed a co-immunoprecipitation assay and confirmed the physical interaction between NFIL3 and T-bet ( Fig. 5g and Supplementary Fig. 12b ). In addition, we performed a competition ChIP-qPCR experiment by preclearing the chromatin sample with antibodies to NFIL3, or control IgG before T-bet ChIP, we found that NFIL3-preclearance attenuates T-bet ChIP at most of the identified T-bet-binding sites in the Tim-3 locus ( Supplementary Fig. 6c ), suggesting the physical interaction between T-bet and NFIL3 that we identified in co-immunoprecipitation (co-IP) represents true binding of NFIL3 and T-bet to the Tim-3 locus. Taken together, our data indicate that IL-27-enhanced Tim-3 expression in Th1 cells is dependent on the combinatorial action of NFIL3 and T-bet in remodelling the Tim-3 locus. We further performed computational analysis of approximately 40 kb of genomic DNA sequence in the mouse Tim-3 locus aligned with the human homologous sequence. We identified conserved non-coding sequences (CNSs) located in the distal and proximal promoter regions (CNSs 6, 12, 13) as well as introns 1 and 5 (CNSs 15, 28) that contain putative NFIL3-binding sites. In ChIP-qPCR analysis, these regions exhibited significantly higher enrichment of NFIL3 binding in WT cells than in NFIL3 −/− cells ( Fig. 5f and Supplementary Fig. 7 ), suggesting that the cis -regulatory function of NFIL3 may also be critical for human Tim-3 transcription. Role of NFIL3 in gut inflammation Our data indicate that IL-27-induced NFIL3 plays a key role in the induction of Tim-3 and IL-10 in effector T cells and increases dysfunctional phenotype in effector CD4 + T cells. We therefore hypothesized that overexpression of NFIL3 could dampen effector T-cell function. Thus, we transduced naïve CD4 + T cells with NFIL3-expressing retrovirus (NFIL3) and transferred these cells into Rag1 −/− (ref. 13 ) recipient mice and observed these mice for the development of gut inflammation. Recipient mice that received NFIL3-transduced CD4 + T cells failed to develop wasting disease 10 weeks after transfer ( Fig. 6a ), when compared with the control mice that received empty virus-transduced (GFP) CD4 + T cells. Histological analysis further revealed that empty virus-transduced T cells induced significantly higher mucosal inflammation than NFIL3-transduced T cells. After grading the crypt damage and cell infiltration (as described in Supplementary Fig. 8a ), we observed that almost all of the recipient mice that received empty virus-transduced CD4 + T cells developed clear histological signs of both enteritis and colitis. In contrast, about half of the mice transferred with NFIL3-transduced T cells did not have any signs of gut inflammation and the rest of the mice had a milder inflammation when compared with the mice transferred with control empty virus-transduced T cells ( Fig. 6b ). We also found that NFIL3-transduced T cells were localized in Peyer’s patches, suggesting that failure to induce inflammation in the gut was not due to a defect of cell migration ( Supplementary Fig. 8b ). In addition, when we harvested empty virus- and NFIL3-transduced cells from the mesenteric lymph nodes of recipient mice 6 weeks post transfer, we found that NFIL3-transduced cells exhibited high Tim-3 expression and IL-10 production, but low IFN-γ production. Although not statistically significant, a clear trend towards low IL-2 production was also observed ( Fig. 6c ). Collectively, these data indicate that the effector function of NFIL3-transduced CD4 + T cells was suppressed in vivo , thereby attenuating the induction of gut inflammation. 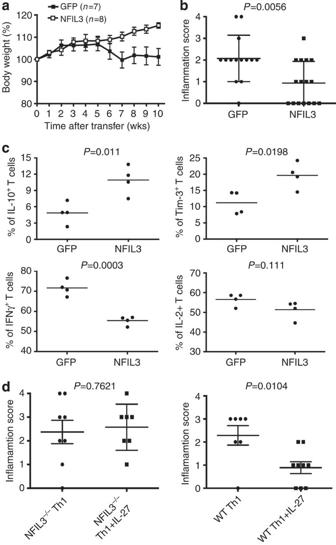Figure 6: Ectopic expression of NFIL3 in CD4+T cells attenuates gut pathology in adoptively transferred enteritis/colitis. Naïve CD4+T cells from C57BL/6 mice were transduced with NFIL3-expressing retrovirus (NFIL3) or control empty retrovirus (GFP). Cells were injected intraperitoneally (i.p.) into Rag1−/−recipient mice to induce gut inflammation (0.7 × 107cells per mouse). (a) Wasting disease was monitored for 10 weeks after transfer. Statistical analysis was performed on the combination of total animals from two independent experiments. Data are shown as mean±s.e.m. Mann–Whitney test two-tailedP=0.0064. (b) Immunopathology of gut inflammation. Two randomly selected tissue sections from each animal were graded for crypt damage and T-cell infiltration. Two scores were given to each animal to represent the overall gut immunopathology. Data are shown as mean±s.e.m. Unpairedt-test two-tailedP=0.0056. (c) The recipient mice were killed 6 weeks after T-cell transfer forex vivoanalysis of cytokine production (IL-2, IL-10 and IFN-γ) and Tim-3 expression by flow cytometry. (d) Naïve CD4+T cells fromWT FoxP3-GFP KIandNFIL3−/−x FoxP3-GFP KImice (CD4+CD62L+GFP−) were differentiated into Th1 cells with or without the presence of IL-27. On day 6, GFP+(FoxP3+) cells were isolated by cell sorting and were injected i.p. intoRag1−/−recipients to induce colitis. Colon pathology was analysed 8 weeks after transfer. Each score represents the pathology from one recipient mouse (NFIL3−/−Th1n=8;NFIL3−/−Th1+IL-27n=7;WTTh1n=7;WTTh1+IL-27n=9. Data are shown as mean±s.e.m.,t-test). Figure 6: Ectopic expression of NFIL3 in CD4 + T cells attenuates gut pathology in adoptively transferred enteritis/colitis. Naïve CD4 + T cells from C57BL/6 mice were transduced with NFIL3-expressing retrovirus (NFIL3) or control empty retrovirus (GFP). Cells were injected intraperitoneally (i.p.) into Rag1 −/− recipient mice to induce gut inflammation (0.7 × 10 7 cells per mouse). ( a ) Wasting disease was monitored for 10 weeks after transfer. Statistical analysis was performed on the combination of total animals from two independent experiments. Data are shown as mean±s.e.m. Mann–Whitney test two-tailed P =0.0064. ( b ) Immunopathology of gut inflammation. Two randomly selected tissue sections from each animal were graded for crypt damage and T-cell infiltration. Two scores were given to each animal to represent the overall gut immunopathology. Data are shown as mean±s.e.m. Unpaired t -test two-tailed P =0.0056. ( c ) The recipient mice were killed 6 weeks after T-cell transfer for ex vivo analysis of cytokine production (IL-2, IL-10 and IFN-γ) and Tim-3 expression by flow cytometry. ( d ) Naïve CD4 + T cells from WT FoxP3-GFP KI and NFIL3 −/− x FoxP3-GFP KI mice (CD4 + CD62L + GFP − ) were differentiated into Th1 cells with or without the presence of IL-27. On day 6, GFP + (FoxP3 + ) cells were isolated by cell sorting and were injected i.p. into Rag1 −/− recipients to induce colitis. Colon pathology was analysed 8 weeks after transfer. Each score represents the pathology from one recipient mouse ( NFIL3 −/− Th1 n =8; NFIL3 −/− Th1+IL-27 n =7; WT Th1 n =7; WT Th1+IL-27 n =9. Data are shown as mean±s.e.m., t -test). Full size image We further addressed the role of IL-27-driven NFIL3 in regulating Th1-driven gut inflammation. For this, we crossed NFIL3 −/− mice to FoxP3-GFP KI mice. We then differentiated the CD4 + CD62L + FoxP3 − (GFP − ) cells from NFIL3 −/− x FoxP3 KI and WT FoxP3 KI mice into Th1 effector cells with or without IL-27 and transferred the cells into Rag1 −/− mice to induce colitis. Mice that received WT Th1 cells showed clear signs of T-cell infiltration and tissue damage, but IL-27-treated WT Th1 cells were much less colitogenic. By contrast, both NFIL3 −/− Th1 cells and IL-27-treated NFIL3 −/− Th1 cells induced similar degrees of colonic inflammation. IL-27 treatment failed to suppress the pathogenicity of these cells in the absence of NFIL3 ( Fig. 6d , and Supplementary Fig. 9a ). Such IL-27-mediated regulatory effect seems to be associated with elevated expression of Tim-3 in IL-27-treated WT Th1 cells, which is abrogated in the absence of NFIL3 ( Supplementary Fig 9b ). Although, we did not find significantly elevated IL-10 production from IL-27-treated WT Th1 cells ( Supplementary Fig. 9b ). A clear trend of IL-10 induction by IL-27 in WT Th1 cells was detected. Taken together, our data indicate that IL-27 can directly suppress Th1 cell-mediated colitis, and NFIL3 is essential for such regulatory effect. IL-27R-deficient mice are resistant to tumour growth Our in vitro studies identified a potential mechanism by which IL-27 induces the expression of Tim-3 through upregulation of NFIL3 and T-bet. Tim-3 has a critical role in the development of exhausted T cells in chronic diseases such as cancer and chronic viral infection [6] , [7] , [8] , [24] , [25] . We therefore reasoned that the IL-27 signalling pathway may also play a key role in regulating effector T-cell phenotype in chronic diseases. To examine this, we implanted B16F10 melanoma into WSX-1 −/− ( IL-27R −/− ) and wild-type C57BL/6 ( WT ) mice, and monitored tumour growth. WSX-1 −/− mice exhibited reduced tumour burden ( Fig. 7a ) and tumour-infiltrating lymphocytes (TILs) from these mice exhibited significantly reduced NFIL3 expression ( Fig. 7b ). Moreover, compared with WT mice, WSX-1 −/− mice failed to develop Tim-3 + PD-1 + T cells, which we have previously identified as the most exhausted T-cell population among TILs [6] ( Fig. 7c ). Indeed, the CD8 + T cells from WSX-1 −/− mice did not exhibit exhausted phenotype, but rather produced more IL-2, IFN-γ and TNF than CD8 + T cells from WT recipient mice ( Fig. 7d ). Importantly, resistance to tumour growth and failure to develop Tim-3 + PD-1 + TILs is also observed in WSX-1 −/− mice bearing Lewis Lung carcinoma ( Supplementary Fig. 10 ). 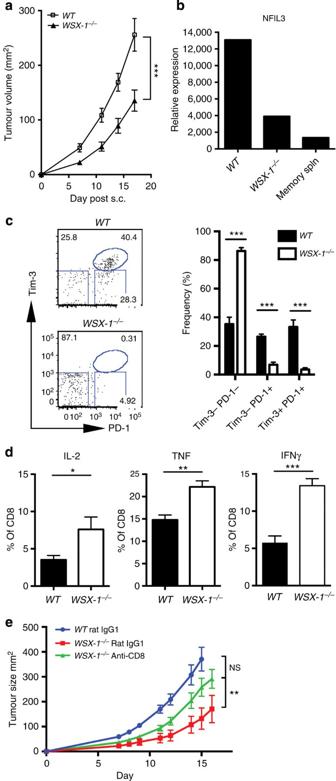Figure 7: IL-27R-deficient mice (WSX-1−/−) are resistant to tumour growth. (a) B16F10 melanoma cells were implanted into C57BL/6 (WT) andWSX-1−/−mice and tumour growth was monitored in two dimensions by caliper as the product of two perpendicular diameters. Statistics was based on combination of total animals from two independent experiments (WT:n=16;WSX-1−/−:n=14. Data are shown as mean±s.e.m.,P<0.0001, linear regression.). (b) Tumour-infiltrating lymphoctyes (TILs) from these mice were isolated and were subjected to reverse transcription–quantitative PCR analysis for NFIL3 expression. (c) The expression of Tim-3 and PD-1 on CD8+TILs fromWT(n=5) andWSX-1−/−(n=5) recipient tumour-bearing mice was determined by flow cytometry. Tim-3−PD-1−:P<0.0001; Tim-3−PD-1+:P<0.0001; Tim-3+PD-1+:P=0.0004,t-test. (d) Production of IL-2, IFN-γ and TNF from peripheral CD8+T cells fromWTandWSX-1−/−mice was determined by flow cytometry. Data are representative of at least two independent experiments with similar results (b,candd: mean±s.e.m. IL-2:P=0.013; TNF:P=0.0012; IFNγ:P=0.0002,t-test). (e)WTandWSX-1−/−mice were implanted with 5 × 105B16F10 tumour cells. On days 1, 2, 8 and 9, 100 μg of anti-CD8 antibody (53-5.8) or Rat IgG1 was injected intraperitoneally. Tumour growth was monitored in two dimensions by caliper (WT:n=9;WSX-1−/−Rat IgG1:n=7;WSX-1−/−Anti-CD8:n=9;P=0.0021, linear regression). Figure 7: IL-27R-deficient mice ( WSX-1 −/− ) are resistant to tumour growth. ( a ) B16F10 melanoma cells were implanted into C57BL/6 ( WT ) and WSX-1 −/− mice and tumour growth was monitored in two dimensions by caliper as the product of two perpendicular diameters. Statistics was based on combination of total animals from two independent experiments ( WT : n =16; WSX-1 −/− : n =14. Data are shown as mean±s.e.m., P <0.0001, linear regression.). ( b ) Tumour-infiltrating lymphoctyes (TILs) from these mice were isolated and were subjected to reverse transcription–quantitative PCR analysis for NFIL3 expression. ( c ) The expression of Tim-3 and PD-1 on CD8 + TILs from WT ( n =5) and WSX-1 −/− ( n =5) recipient tumour-bearing mice was determined by flow cytometry. Tim-3 − PD-1 − : P <0.0001; Tim-3 − PD-1 + : P <0.0001; Tim-3 + PD-1 + : P =0.0004, t -test. ( d ) Production of IL-2, IFN-γ and TNF from peripheral CD8 + T cells from WT and WSX-1 −/− mice was determined by flow cytometry. Data are representative of at least two independent experiments with similar results ( b , c and d : mean±s.e.m. IL-2: P =0.013; TNF: P =0.0012; IFNγ: P =0.0002, t -test). ( e ) WT and WSX-1 −/− mice were implanted with 5 × 10 5 B16F10 tumour cells. On days 1, 2, 8 and 9, 100 μg of anti-CD8 antibody (53-5.8) or Rat IgG1 was injected intraperitoneally. Tumour growth was monitored in two dimensions by caliper ( WT : n =9; WSX-1 −/− Rat IgG1: n =7; WSX-1 −/− Anti-CD8: n =9; P =0.0021, linear regression). Full size image To determine whether the reduced tumour growth in WSX-1 −/− mice is CD8 + T-cell dependent, we depleted CD8 + T cells in mice implanted with B16F10 melanoma. Isotype rat IgG treatment in WSX-1 −/− and in WT mice did not alter the phenotypic difference in tumour growth as we found in previous experiments. By contrast, CD8 + T-cell depletion in WSX-1 −/− mice significantly accelerated tumour growth and abrogated the protective effects of WSX-1 deficiency ( Fig. 7e ). Together, these data indicate that IL-27 signalling is critical for the induction of NFIL3 and Tim-3 expression and mediating T-cell dysfunction in cancer. We further addressed the role of NFIL3 in tumour growth. For this, we transferred wild-type or NFIL3 −/− T cells into Rag1 −/− mice, and subsequently inoculated with B16F10 melanoma cells. We found that tumour growth in NFIL3 −/− T-cell recipient mice was significantly delayed ( Supplementary Fig. 11a,b ) and that Tim-3 expression on CD4 + TILs was significantly reduced compared with WT . Interestingly, we did not see large defects in Tim-3 expression on CD8 + TILs ( Supplementary Fig. 11c ). These data suggest that Tim-3 expression on CD8 + TILs is relatively less NFIL3-dependent compared with CD4 + TILs. This likely reflects functional redundancy by other transcriptional factors that are induced in the tumour environment to drive Tim-3 expression in CD8 + T cells. It has been well established that interaction between Tim-3 and its ligand galectin-9 inhibits Th1 responses [9] , [26] , [27] and induces peripheral tolerance [28] , [29] . More importantly, Tim-3 is now recognized as having a key role in the induction of T-cell exhaustion during chronic viral infections. Blockade of Tim-3 enhances proliferation and cytokine production in both HIV-1- and HCV-specific CD8 + T cells [3] , [30] . Similarly, blockade of Tim-3 signalling also improves functional responses in TILs in cancers [6] , [7] , [8] . In contrast, a reduction in the expression of Tim-3 has been associated with the development of autoimmune diseases [13] . These observations highlight the role of Tim-3 in regulating T-cell effector function in chronic diseases and underscore the need for elucidating how Tim-3 expression is regulated. We report that the immunosuppressive cytokine IL-27 sets in motion the Tim-3-dependent transcriptional programme of T-cell inhibition. IL-27 induces expression of the transcription factor NFIL3, which co-regulates the expression of both Tim-3 and IL-10, two molecules associated with dysfunctional T cells. T-bet is the first transcription factor directly linked to Tim-3 transcription. Although multiple studies showed that Tim-3 + exhausted T cells proportionally express high amounts of T-bet [3] , [31] , the role of T-bet in regulating Tim-3 was contradictory. For example, although T-bet transgenic T cells exhibited enhanced Tim-3 expression [14] , T cells with retrovirally transduced with T-bet exhibited slightly reduced Tim-3 expression during chronic LCMV infection [19] . Taken together, these observations raised doubt as to whether T-bet alone is sufficient to drive Tim-3 expression, and pointed to the possibility that additional mechanisms may be involved in both the induction of Tim-3 and T-cell dysfunction. Here, we have identified the anti-inflammatory cytokine IL-27 as a potent signal for Tim-3 induction in T cells. In addition, we characterize a molecular mechanism by which the IL-27-triggered signal cascade directly controls the transcription of Tim-3 expression via STAT3-dependent induction of NFIL3 and also via STAT1-dependent induction of T-bet. Our findings further indicate that the STAT3-NFIL3 pathway is the key pathway in the induction of Tim-3 and largely explains the potency of IL-27 in the induction of Tim-3. Importantly, NFIL3 exhibited a direct dose-dependent effect on the induction of Tim-3 expression, and as such further cooperates with T-bet to induce Tim-3 expression. These observations support our hypothesis that T-bet is necessary but not sufficient for Tim-3 transcriptional activity and that NFIL3 is the key transcription factor that collaborates with T-bet to induce optimal Tim-3 expression. IL-27 has been reported to act as an anti-inflammatory cytokine in multiple disease settings: autoimmune diseases [32] , [33] , [34] , bacterial infections [35] , [36] and acute viral infections [8] . Among the molecular mechanisms implicated in the anti-inflammatory effects of IL-27 are those that block differentiation of naïve T cells into Th2 and Th17 cells by IL-27 targeting their master transcription factors RORγt [37] and GATA3 (ref. 38 ). In addition to suppressing the transcriptional programme for effector T-cell differentiation, a recent study indicated that IL-27 directly induces expression of inhibitory molecules like PD-L1 (ref. 39 ). Together with our data showing that IL-27 induces Tim-3, these data indicate that induction of inhibitory molecules associated with T-cell dysfunction in T cells might be another mechanism by which IL-27 mediates its inhibitory effects. Although in vitro stimulation with IL-27 has been shown to promote Th1 differentiation [17] and augment cytotoxic T lymphocyte function [40] , there are also data showing that IL-27 suppresses both effector Th1 and Tc1 responses through induction of IL-10 expression [41] , [42] . Our data support that IL-27 controls immune responses by at least two different mechanisms: (i) by inducing IL-10 production and (ii) by inducing inhibitory molecules such as Tim-3 and PD-L1 on differentiated effector Th1 and Tc1 cells, thus promoting T-cell dysfunction. Indeed, we have demonstrated in the current study that: (i) IL-27-conditioned Th1 cells induce less severe colitis and (ii) endogenous IL-27 signalling results in reduced tumour burden because of enhanced effector CD8 function that is associated with increased proinflammatory cytokine production and reduced expression of Tim-3 and PD-1 in TILs. In conclusion, our data indicate a key role for IL-27 in the regulation of T-cell dysfunction. Thus, targeting the IL-27 pathway could be of value as a therapeutic strategy in cancer and other chronic diseases. NFIL3 is a key suppressor of IL-12 p40 gene expression in macrophages [43] , therefore it negatively regulates innate immunity. Similarly, its anti-inflammatory role in the regulation of adaptive immune responses has been appreciated, in that NFIL3 was shown to induce IL-10 production in multiple T-cell subsets [21] , [44] . NFIL3 −/− effector T cells exhibit reduced IL-10 production, and exhibit severe defect in controlling effector function thereby resulting in more severe CNS autoimmunity and colitis [21] . Consistent with these data, our current study shows that forced expression of NFIL3 in T cells suppresses their effector function and significantly reduces gut pathology in RAG-deficient recipient mice. Importantly, a previous study showed that STAT3 is a major transducer for IL-27-mediated suppression of cytokine production [45] . As the induction of NFIL3 by IL-27 signalling is STAT3 dependent, our data strongly indicate that NFIL3 is an important functional mediator of the IL-27-driven anti-inflammatory effect by inducing Tim-3 and IL-10 expression and rendering T cells dysfunctional. Such NFIL3-dependent mechanism in IL-27-induced Tim-3 expression has been well validated in effector CD4 + T cells in both colitis and tumour models. Interestingly, the induction of Tim-3 is not significantly affected in NFIL3 −/− CD8 + TILs, suggesting that a redundant downstream pathway in IL-27 signalling might compensate for lack of NFIL3 in CD8 + T cells. This could also reflect extreme pressure in the tumour microenvironment to drive Tim-3 expression and T-cell dysfunction in CD8 + T cells. Nevertheless, our data also indicate that the IL-27-NFIL3 axis has an important role in the regulation of T helper cells in anti-tumour immunity. In summary, we provide evidence supporting that IL-27 is a critical anti-inflammatory cytokine that induces the transcription factor NFIL3, whose function is essential for the development of dysfunctional T-cell phenotype: high Tim-3 and IL-10, and low IL-2 and IFN-γ. As such, our observations place the IL-27 signalling pathway upstream of the suppression programme that drives the development of T-cell dysfunction in cancer. Consequently, blockade of IL-27 signalling may be a highly effective means by which T-cell dysfunction could be abrogated for the treatment of cancer and other chronic diseases where T-cell exhaustion is a barrier in mounting an effective immune response. Mice STAT1 −/− mice and 129S wild-type mice were purchased from Taconic. Rag1 −/− mice, T-bet −/− mice and C57BL/6 mice were purchased from the Jackson Laboratory. Peripheral lymphoid organs from STAT3 fl/fl x CD4-Cre ( STAT3 cko ) mice and STAT3 fl/fl control mice were provided by Dr John O’Shea at the National Institutes of Health. NFIL3 −/− mice were provided by Dr Tak Mak at the University of Toronto. WSX-1 −/− mice were provided by Dr Chris Saris at Amgen. WT FoxP3-GFP KI and NFIL3 −/− x FoxP3-GFP KI mice are bred in house. All mice were bred and kept in pathogen-free barriers. In vivo animal experiments were done using 7- to 8-week-old female mice. Protocols for animal studies were approved by the Institutional Animal Care and Use Committee at the Harvard Medical School. Antibodies and cytokines The following antibodies for T cells surface staining and flow cytometry were purchased from BioLegend: phycoerythrin-indotricarbocyanine (PE)-anti-CD4 (clone RM4-5), allophycocyanin (APC)-anti-CD62L (clone MEL-14), PE-anti-CD8 (clone 53-6.7), anti-IL-10 (clone JES5-16E3), anti-TNF (clone TN3-19.12), anti-IL-2 (clone JES6-5H4), anti-IFN-γ (clone XMG1.2), APC-LAG3 (clone C9B7W), PE-anti-PD-1 (RMP1–30). PE-anti-CD90.1 (clone OX-7). PE-anti-CD160 (clone eBioCNX46.3) was purchased from eBioscience. APC-anti-Tim-3 (5D12) was prepared in house. Antibodies were diluted 200 times for cell staining. All of the recombinant mouse cytokines for T-cell in vitro culture and Tim-3 induction were purchased from R&D systems. Cell isolation and culture Total CD4 + T cells from different lines of mice were first enriched by positive selection using CD4 + T-cell isolation reagent from Miltenyi Biotec. Naïve CD4 + (CD4 + CD62L + ) T cells were stained by PE-anti-CD4 and APC-anti-62L antibodies and were subsequently sorted by BD FACSAria (BD Biosciences). The sorted naïve T cells were then activated with plate-bound anti-CD3 (1 μg ml −1 ; 145-2C11) and anti-CD28 (1 μg ml −1 ; PV-1; both were made in house) for 2 days and were rested afterwards in the presence of 10 ng ml −1 of IL-2. Th1 cells were cultured under the presence of IL-12 (10 ng ml −1 ). In some conditions, 25 ng ml −1 of IL-27 were added. Gene expression profiling Naïve CD4 + T cells were activated with anti-CD3 and anti-CD28 antibodies with or without the presence of IL-27 for 60 h. Total RNA was isolated with an RNeasy Plus kit (Qiagen) and then was amplified with an Ovation Biotin RNA Amplification and Labeling System (NuGEN). The complementary DNA (10 μg) was fragmented and labelled and then was hybridized to a GeneChip Mouse Genome 430 2.0 array (Affymetrix). Comparative gene expression between Th0 and IL-27-treated CD4 + T cells was analysed by GenePattern software. The data have been deposited in NCBI Gene Expression Omnibus (GEO) under the accession code GSE63628. Retroviral transduction cDNAs encoding mouse NFIL3 and T-bet were subcloned into modified pMSCV vector that bicistronically expresses GFP (for NFIL3), and Thy1.1 (for Thy1.1), respectively. Retroviruses were packed in 293 T cells and were used to transduce mouse naïve CD4 + T cells activated by plate-bound anti-CD3 and anti-CD28 antibodies. Intracellular cytokine staining Naïve CD4 + T cells were activated by plate-bound anti-CD3 and anti-CD28 antibodies for 2 days. Cells were then rested for 3 days in the presence of 10 ng ml −1 of IL-2, and restimulated with 0.1 μg ml −1 of plate-bound anti-CD3 and anti-CD28 for 24 h before they were subjected to phorbol myristate acetate and ionomycin stimulation in the presence of Golgi Stop (BD Biosciences) for intracellular cytokine detection. All data were collected on LSR II (BD Biosciences) or Calibor (BD Biosciences) and analysed by FlowJo software (Tree Star, Inc.). ChIP assays Naïve CD4 + T cells from C57BL/6 mice were purified by naïve CD4 + T cell-negative selection kit (Miltenyi Biotec), and were activated by plate-bound anti-CD3 and anti-CD28 (2 μg ml −1 each) under either neutral condition (Th0) or Th1 differentiating condition in the presence of IL-27 (Th1+IL-27) for 2 days. Cells were rested for additional 3 days in the presence of 10 ng ml −1 of IL-2 and were restimulated with 0.1 μg ml −1 of plate-bound anti-CD3 and anti-CD28 for 24 h before they were subjected to chromatin preparation for the ChIP analysis. Chromatin fraction preparation and chromatin IP were performed using SimpleChIP Enzymatic Chromatin IP Kit (Cell Signaling Technology). Antibody against NFIL3 (C-18) was purchased from Santa Cruz Biotechnology, anti-acetylated Histone 3 antibody (Cat# 06-599) was purchased from Millipore and an anti-trimethylated Histone Lysine 4 antibody (Cat# ab8580) was purchased from Abcam. Real-time PCR analysis RNA was extracted with RNeasy Plus kits (Qiagen) and cDNA was made by Iscript (Bio-Rad). All of the real-time PCR probes were purchased from Applied Biosystems. QPCR were performed by the GeneAmp7500 Sequence Detection System and ViiA7 Real-Time PCR System (Applied Biosystems). Tumour challenge and phenotypic/functional studies B16F10 melanoma (CRL-6475) cell line was purchased from ATCC. 5 × 10 5 cells were injected subcutaneously at the flanks of the mice. Tumours were measured in two dimensions using caliper as the product of two perpendicular diameters. TILs were isolated on day 14 to day 20 post tumour implantation as they were reaching 200 mm 2 in size [6] . Single-cell suspensions were stained for CD8, CD4, Tim-3 and PD-1. For functional assay, intracellular cytokine staining was conducted as described before [6] . For gene expression analysis, CD8 + 7AAD − TILs of B16 melanoma on WT C57BL/c mice or WSX-1 −/− mice were sorted by BD FACSAria after magnetic separation by Dynabeads FlowComp Mouse CD8 (Invitrogen). CD44 hi CD62L low memory CD8 + splenocytes from B6 non-tumour-bearing mice were also sorted as a control. RNA from sorted CD8 + cells were then extracted and reverse transcribed to cDNA. Gene expressions were quantified by qPCR. Gut pathology Naïve CD4 + T cells from C57BL/6 mice were subjected to TcR activation by anti-CD3 and anti-CD28 antibodies. Cells were subsequently transduced with NFIL3-expressing retrovirus or GFP-expressing empty retrovirus in the next day. On day 5 after activation, GFP-positive T cells were sorted by BD FACSAria (BD Biosciences) and were transferred intraperitoneally into Rag1 −/− recipient mice. To analyse Tim-3 expression and cytokine production, NFIL3- or GFP-transduced cells were intraperitoneally injected to Rag1 −/− mice. Mice were killed 6 weeks after injection. Cells from spleen and mesenteric lymph nodes were restimulated with PMA/ionomycin in the presence of Golgi Stop (BD Biosciences) for detection of cytokine production and Tim-3 expression by flow cytometry. Body weight and symptoms of disease were monitored up to 10 weeks. At the end point of the experiment, mice were killed. Intestines were fixed with 10% formalin and sections were stained with haematoxylin and eosin. The slides were evaluated independently by Dr Vijay Yajnik at the Massachusetts General Hospital and Dr Roderick Bronson at the Rodent Histopathology Core, Harvard Medical School. Additional transfer colitis was performed using naïve CD4 + T cells from WT FoxP3-GFP KI and NFIL3 −/− x FoxP3-GFP KI mice (CD4 + CD62L + GFP − ) that were activated by plate-bound anti-CD3/CD28 in the presence of 10 ng ml −1 of IL-12, 10 μg ml −1 of anti-TGFβ1-2-3 antibody and 10 μg ml −1 of anti-IL-4 antibody. The cells were simultaneously treated with or without 25 ng ml −1 of IL-27. On day 6, cells were sorted again to deplete GFP + (FoxP3 + ) cells, and were peritoneally injected into Rag1 −/− recipients (0.6 × 10 6 cells per mouse) to induce colitis. How to cite this article : Zhu, C. et al. An IL-27/NFIL3 signalling axis drives Tim-3 and IL-10 expression and T-cell dysfunction. Nat. Commun. 6:6072 doi: 10.1038/ncomms7072 (2015).